Identity of aPlasmodiumlactate/H+symporter structurally unrelated to human transporters Maintenance of a high glycolytic flow rate is critical for the rapid growth and virulence of malarial parasites. The parasites release two moles of lactic acid per mole of glucose as the anaerobic end product. However, the molecular identity of the Plasmodium lactate transporter is unknown. Here we show that a member of the microbial formate–nitrite transporter family, PfFNT, acts as a lactate/proton symporter in Plasmodium falciparum . Besides L -lactate, PfFNT transports physiologically relevant D -lactate, as well as pyruvate, acetate and formate, and is inhibited by the antiplasmodial compounds phloretin, furosemide and cinnamate derivatives, but not by p -chloromercuribenzene sulfonate (pCMBS). Our data on PfFNT monocarboxylate transport are consistent with those obtained with living parasites. Moreover, PfFNT is the only transporter of the plasmodial glycolytic pathway for which structure information is available from crystals of homologous proteins, rendering it amenable to further evaluation as a novel antimalarial drug target. Glucose is the prime energy source of malarial parasites [1] . Erythrocytes infected with Plasmodium spp. consume glucose up to two orders of magnitude faster than uninfected cells, generating lactic acid as the anaerobic end product [1] . Glucose uptake from the host serum is facilitated by the erythrocyte glucose transporter 1 (ref. 2 ), and, consecutively, by the plasmodial hexose transporter (HT) [3] . Erythrocytes release lactic acid into the blood via a lactate/proton symporter Monocarboxylate Transporter 1 (MCT1) [4] and parasite-induced permeation pathways [5] . Until today, the parasite’s lactate transporter has escaped discovery. The abundance of glucose in the host blood allows the parasites to thrive rapidly despite inefficient energy generation by anaerobic glycolysis ( Fig. 1a ). Glycolytic oxidation of D -glucose to pyruvate concomitantly converts NAD + to NADH, which is recycled by lactate dehydrogenase-catalysed reduction of pyruvate to L -lactate. In total, per mole of glucose, plasmodia generate 2 moles each of ATP, lactate and protons. The steady state is, hence, characterized by high rates of glucose influx and twice as high rates of lactate and proton efflux (18 mmol l –1 min –1 ) [6] . Therefore, the glucose and lactate transporters are considered valuable drug targets [7] , [8] , provided that their protein structures differ sufficiently from their human counterparts for selectivity reasons. 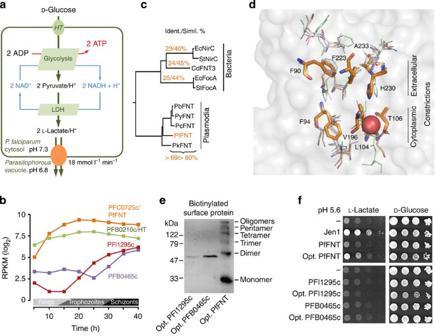Figure 1: Identification of PfFNT as a plasmodial lactate transporter. (a) Glycolytic flow in malarial parasites with the molecular identity of the lactate/proton symporter unknown (HT, hexose transporter; LDH, lactate dehydrogenase). (b) Expression profile of the plasmodial HT (green) and candidate lactate transporters PFB0465c (purple), PFI1295c (red) and PfFNT (orange). Data were from plasmoDB10,11; transcript level is given as reads per kilobase of exon model per million mapped reads (RPKM)11. (c) Identity and similarity of PfFNT (orange) to other plasmodial (Pb,P. berghei; Py,P. yoelii; Pc,P. chabaudi; Pk,P. knowlesi) and bacterial FNTs (Ec,Escherichia coli; St,Salmonella typhimurium, Cd,Clostridium difficile). (d) Side view on the EcFocA12,14(green), StNirC15(pink) and CdFNT3 (ref.17; blue) structures plus a PfFNT model (orange). Depicted are residues of the transport channel with the constriction sites as sticks and a fixed water molecule (red sphere). (e) Western blot showing plasma membrane localization of codon-optimized PfFNT, PFI1295c and PFB0465c in yeast. (f) Growth phenotype of yeast without endogenous lactate transporters (jen1Δady2Δ)19. Growth onL-lactate as the sole carbon source indicates lactate transport of the expressed protein. Figure 1: Identification of PfFNT as a plasmodial lactate transporter. ( a ) Glycolytic flow in malarial parasites with the molecular identity of the lactate/proton symporter unknown (HT, hexose transporter; LDH, lactate dehydrogenase). ( b ) Expression profile of the plasmodial HT (green) and candidate lactate transporters PFB0465c (purple), PFI1295c (red) and PfFNT (orange). Data were from plasmoDB [10] , [11] ; transcript level is given as reads per kilobase of exon model per million mapped reads (RPKM) [11] . ( c ) Identity and similarity of PfFNT (orange) to other plasmodial (Pb, P. berghei ; Py, P. yoelii ; Pc, P. chabaudi ; Pk, P. knowlesi ) and bacterial FNTs (Ec, Escherichia coli ; St, Salmonella typhimurium , Cd, Clostridium difficile ). ( d ) Side view on the EcFocA [12] , [14] (green), StNirC [15] (pink) and CdFNT3 (ref. 17 ; blue) structures plus a PfFNT model (orange). Depicted are residues of the transport channel with the constriction sites as sticks and a fixed water molecule (red sphere). ( e ) Western blot showing plasma membrane localization of codon-optimized PfFNT, PFI1295c and PFB0465c in yeast. ( f ) Growth phenotype of yeast without endogenous lactate transporters ( jen1 Δ ady2 Δ) [19] . Growth on L -lactate as the sole carbon source indicates lactate transport of the expressed protein. Full size image The plasmodial HT has been cloned and biochemically characterized, and first inhibitors have shown antimalarial potential [9] . Plasmodial lactate transport has been characterized using living parasites and revealed a low-affinity and high-capacity lactate/proton symport mechanism [5] , [7] , [8] . The P. falciparum genome encodes two proteins (PFB0465c, 51.9 kDa and PFI1295c, 60.7 kDa) [10] , which are reminiscent of human monocarboxylate transporters with respect to sequence similarity and predicted topology ( Supplementary Figs 1 and 2 , Supplementary Table 1 ). However, the mRNA levels are low and the expression profiles during the intraerythrocytic parasite development neither correlate with that of the HT nor with the respective metabolic activity ( Fig. 1b ) [10] , [11] . PFB0465c and PFI1295c expression is maximal at the late schizont stage when merozoites are formed, whereas the HT peaks at the metabolically most active trophozoite stage and then remains high. In this study, we show the molecular identity of a plasmodial lactate/proton symporter (PFC0725c) whose properties match those obtained with living parasites before. The expression profile of PFC0725c is linked to glycolysis PFC0725c encodes a single putative formate–nitrite transporter (PfFNT, 34.4 kDa) whose expression profile [11] , [12] parallels that of the plasmodial HT ( Fig. 1b ), the lactate dehydrogenase and all glycolytic enzymes ( Supplementary Fig. 3 ). Single FNT genes are present throughout the Plasmodium species and code for a protein subfamily with at least 69% sequence identity and 80% similarity ( Fig. 1c , Supplementary Fig. 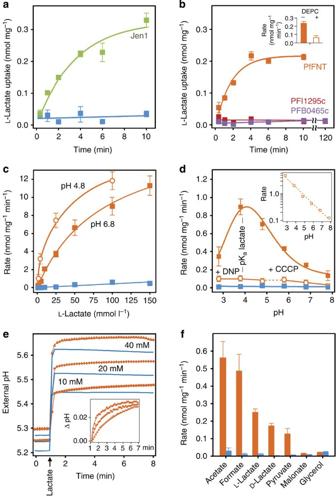Figure 2: Biochemical characterization of plasmodial lactate transporter candidates in yeast. (a)L-Lactate uptake ofjen1Δady2Δ yeast19expressing yeast Jen1 (green) or no transporter (blue). (b)L-Lactate uptake after expression of plasmodial PfFNT (orange), PfB0465c (purple) or PFI1295c (red). The bar graph indicates uptake rates via untreated PfFNT and after chemical blockage by DEPC. (c) Concentration dependency of PfFNTL-lactate transport (orange squares: external pH 6.8; open symbols: pH 4.8) versus nonexpressing controls (blue). (d) pH dependency ofL-lactate transport via PfFNT (orange squares; nonexpressing controls: blue). The inset shows correlation of pH and lactate transport after correction for the pH-dependent lactate/lactic acid ratio. Open circles depict transport reduction by proton gradient decouplers (2,4-dinitrophenol, carbonylcyanide-3-chlorophenylhydrazone). (e) Alkalization of the external buffer due to lactate/proton symport in PfFNT-expressing yeast at 10 mM (circles), 20 mM (diamonds) and 40 mM (triangles) inward lactate gradients. The inset depicts the initial, concentration-dependent proton uptake kinetics. (f) PfFNT monocarboxylate selectivity (orange) versus nonexpressing controls (blue) measured injen1Δady2Δ yeast19using various14C-labelled substrates. Throughout, data were normalized to 1 mg of dry yeast; error bars denote s.e.m. from 3 to 6 measurements. 4 and Supplementary Table 2 ). Generally, FNTs are restricted to microorganisms and operate as pentameric, aquaporin-like transporters for formate [12] , [13] , [14] , nitrite [15] and hydrosulfide [16] . Yet, none of these anions have been reported to be relevant in plasmodial metabolism. Recently, a bacterial FNT (FocA) was shown to transport larger monocarboxylate anions including lactate [17] and to switch to monocarboxylate/proton symport below pH 5.7 (ref. 13 ). FNTs neither fit into the group of classical secondary transporters (for example, MCTs) described by the alternate access model [18] because they do not undergo major conformational changes during transport and, thus, keep both access sites open; nor are they strictly channels (for example, aquaporins), because at a surplus of protons this gradient is thought to enable and drive anion/proton symport [15] . We used the available crystal data of various bacterial FNTs [12] , [14] , [15] , [16] to generate a model of the eukaryotic PfFNT ( Supplementary Fig. 5 ). The structures align with sub-Angstrom deviations at two conserved constriction sites ( Fig. 1d ). PfFNT displays identical residues in seven of these critical positions; the final, eighth position harbours a phenylalanine (Phe94) instead of leucine. The constrictions plus a proton relay [15] consisting of a histidine (His230 in PfFNT), a fixed water molecule (red sphere) and a threonine (Thr106) are thought to define selectivity by transient protonation of permeating weak monoacids [15] . PfFNT transports L -lactate Yeast expression of codon-optimized PfFNT, PFB0465c and PFI1295c ( Supplementary Figs 6–8 ) was successful, and the proteins integrated into the plasma membrane ( Fig. 1e and Supplementary Fig. 9 ). PfFNT exhibited considerable detergent resistance revealing a pentameric structure. For phenotypic evaluation we employed yeast devoid of the endogenous lactate transporters, Jen1 and Ady2 (ref. 19 ). This strain is particularly suited for the assay because of a virtually absent background lactate permeability. Accordingly, the yeast was unable to grow on lactate media and expression of Jen1 rescued the growth defect ( Fig. 1f ). PFB0465c and PFI1295c did not enable proliferation, whereas PfFNT permitted pH-dependent growth hinting at lactate/proton symport ( Fig. 1f and Supplementary Fig. 10 ). PfFNT is a lactate/proton symporter Next, we carried out direct transport assays using 14 C-labelled L -lactate ( Fig. 2a,b ). PfFNT-mediated L -lactate transport exhibited an initial rate of 0.25 nmol mg –1 min –1 ( Fig. 2b , inset) similar to Jen1. PFB0465c and PFI1295c did not increase intracellular lactate concentrations even after prolonged exposure of 2 h to compensate for lower expression levels. The lack of functionality may be attributed to the absence of three conserved residues in transmembrane spans 1 and 8, which have been shown to be required for lactate transport by MCT1 ( Supplementary Fig. 1 ). Jen1 is unrelated to MCT-like proteins, of which the yeast genome encodes five members, yet none of these facilitates lactate transport [20] . These and the lactate-impermeable Plasmodium MCT-type proteins could suggest that MCTs assumed lactate transport function later in evolution. PfFNT lactate transport was inhibited by the histidine-modifying agent diethylpyrocarbonate (DEPC, Fig. 2b , inset) and transport was bidirectional ( Supplementary Fig. 11 ). Figure 2: Biochemical characterization of plasmodial lactate transporter candidates in yeast. ( a ) L -Lactate uptake of jen1 Δ ady2 Δ yeast [19] expressing yeast Jen1 (green) or no transporter (blue). ( b ) L -Lactate uptake after expression of plasmodial PfFNT (orange), PfB0465c (purple) or PFI1295c (red). The bar graph indicates uptake rates via untreated PfFNT and after chemical blockage by DEPC. ( c ) Concentration dependency of PfFNT L -lactate transport (orange squares: external pH 6.8; open symbols: pH 4.8) versus nonexpressing controls (blue). ( d ) pH dependency of L -lactate transport via PfFNT (orange squares; nonexpressing controls: blue). The inset shows correlation of pH and lactate transport after correction for the pH-dependent lactate/lactic acid ratio. Open circles depict transport reduction by proton gradient decouplers (2,4-dinitrophenol, carbonylcyanide-3-chlorophenylhydrazone). ( e ) Alkalization of the external buffer due to lactate/proton symport in PfFNT-expressing yeast at 10 mM (circles), 20 mM (diamonds) and 40 mM (triangles) inward lactate gradients. The inset depicts the initial, concentration-dependent proton uptake kinetics. ( f ) PfFNT monocarboxylate selectivity (orange) versus nonexpressing controls (blue) measured in jen1 Δ ady2 Δ yeast [19] using various 14 C-labelled substrates. Throughout, data were normalized to 1 mg of dry yeast; error bars denote s.e.m. from 3 to 6 measurements. Full size image PfFNT transport increased linearly with the L -lactate concentration throughout the physiological, low-millimolar range and saturated above 50 mM ( Fig. 2c , closed symbols). We determined an apparent lactate affinity of 87 mM consistent with data from the homologous Salmonella typhimurium FocA ( k lactate 96 mM) [17] . Data on the affinity of lactate transport in live parasites vary strongly with the assay conditions ranging from 3.8 mM as obtained by pH-shift measurements with isolated parasites [8] to apparently nonsaturable when determined as uptake of radiolabelled lactate into permeabilized, infected erythrocytes [5] . This is reminiscent of affinity determinations of E. coli lactose permease varying 100-fold upon changing the membrane potential, the transmembrane proton gradient or transiting from intact cells to vesicle preparations [21] . Notably, equal to FNTs, a histidine is protonated during transduction [22] . Similarly, when we shifted the external pH from 6.8 to 4.8, the affinity of PfFNT for lactate increased fivefold to 17 mM probably due to a higher level of protonation of His230, whereas the maximal transport rate remained unchanged at 14 nmol mg –1 min –1 ( Fig. 2c , open symbols). There is consistent evidence that malarial parasites transport lactate in symport with protons [5] , [7] , [8] . Likewise, lactate transport via PfFNT increased with acidity and was maximal at pH 3.9, that is, the pK a of lactate ( Fig. 2d ). At this pH, lactate and lactic acid are equimolar. Towards more acidic conditions, the proportion of lactate anions decreases as did the transport rate. The low background membrane diffusion of protonated, neutral lactic acid at acidic pH did not interfere with the assay. Correction for the lactate/lactic acid ratio using the Henderson–Hasselbalch equation showed a direct correlation of pH and lactate transport, suggesting lactate/proton symport in all tested pH situations ( Fig. 2d , inset). Addition of protonophores almost abolished transport ( Fig. 2d ) indicating that the transmembrane proton gradient energizes PfFNT lactate transport. Meaningful data can be obtained only at pH values around or above the protonophore’s pK a , hence the splitting of the data range (2,4-dinitrophenol, pK a 4.0, pH 2.8–4.8; carbonylcyanide-3-chlorophenylhydrazone, pK a 6.09, pH 5.8–8.8) [23] . Uptake of L -lactate into yeast cells coincided with alkalization of the weakly buffered external medium in a concentration-dependent manner directly showing lactate/proton co-transport ( Fig. 2e ). Finally, we blocked the alternative proton uptake route in yeast, that is, the potassium/proton antiporter, by adding external potassium to compensate the transmembrane gradient [24] . Yet, lactate transport remained stable, further consolidating a PfFNT lactate/proton symport mechanism ( Supplementary Fig. 12 ). To exclude any influence of the yeast plasma membrane environment on the functionality and selectivity of PfFNT, we reconstituted cell-free produced and purified PfFNT into proteoliposomes. Exposure to L -lactate buffer resulted in proteoliposome swelling as visualized by a decrease in light scattering, confirming PfFNT functionality as a lactate transporter ( Supplementary Fig. 13 ). Our experiments indicate two properties of PfFNT lactate transport: (a) PfFNT accepts lactate in the anion form, which is protonated during transport probably via the His230-water-Thr106 proton relay, and (b) unlike FocA, PfFNT acts as a lactate/proton co-transporter throughout the neutral-to-acidic pH range. Both features comply with plasmodial physiology. The parasite is situated inside the acidic parasitophorous vacuole ( Fig. 1a ) [6] , which by protonation reduces the proportion of local vacuolar lactate anions; in addition, the residence time of lactate in the parasitophorous vacuole is kept low by rapid release into the blood serum [5] , [6] . The outward gradient of lactate together with the anion selectivity of PfFNT drives transport in the export direction; the symport with protons prevents acidification of the parasite’s cytosol. Owing to the high glycolytic rate, plasmodia produce considerable amounts of toxic methylglyoxal as a nonenzymatic byproduct, which is expelled via the aquaglyceroporin PfAQP [25] , [26] or converted to D -lactate (6–7% of the total lactate) for detoxification and release [27] . Appropriately, PfFNT transported D -lactate among other short-chain monocarboxylates ( Fig. 2f ). The similarly sized dicarboxylate malonate and uncharged glycerol were excluded. Inhibition of PfFNT by small molecules Earlier studies showed that certain compounds, such as phloretin, furosemide and cinnamic acid derivatives, inhibit plasmodial lactate transport [7] , [8] resulting in cell death [28] . Importantly, the organomercurial p -chloromercuribenzene sulfonate (pCMBS), that inhibits human MCTs by convalently modifying their essential ancillary protein, basigin [29] , does not block Plasmodium lactate transport [7] . In our experiments, phloretin, furosemide, α-cyano-4-hydroxy-cinnamate and α-fluorocinnamate inhibited PfFNT with IC 50 values ~1 mM ( Fig. 3a–d ). Inhibition required a negatively charged moiety because the neutral cinnamamide was nonfunctional ( Fig. 3e ). Strikingly in line with the in vivo data, pCMBS did not inhibit PfFNT ( Fig. 3f ). 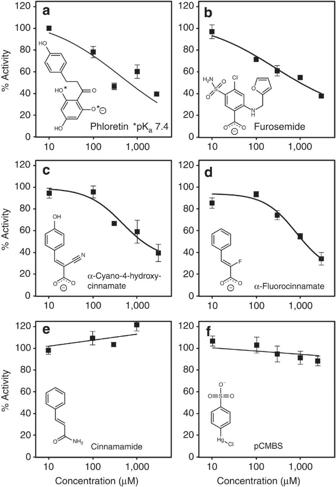Figure 3: Inhibition of PfFNTL-lactate transport. Phloretin (a), furosemide (b) and cinnamic acid derivatives (c,d) inhibit PfFNT, whereas neutral cinnamamide (e) and pCMBS do not (f). Measurements were conducted injen1Δady2Δ yeast19; error bars indicate s.e.m. of triple determinations. Figure 3: Inhibition of PfFNT L -lactate transport. Phloretin ( a ), furosemide ( b ) and cinnamic acid derivatives ( c , d ) inhibit PfFNT, whereas neutral cinnamamide ( e ) and pCMBS do not ( f ). Measurements were conducted in jen1 Δ ady2 Δ yeast [19] ; error bars indicate s.e.m. of triple determinations. Full size image PfFNT resides in the plasmodial plasma membrane Finally, we expressed a PfFNT-GFP (green fluorescent protein) fusion protein for localization in P. falciparum parasites [30] , [31] . Fluorescence was restricted to the intraerythrocytic parasite and concentrated at the parasite’s periphery where it co-localized with the plasma membrane protein merozoite surface protein 1 (MSP1; Fig. 4 ), which is consistent with a function of PfFNT in lactate and proton release. 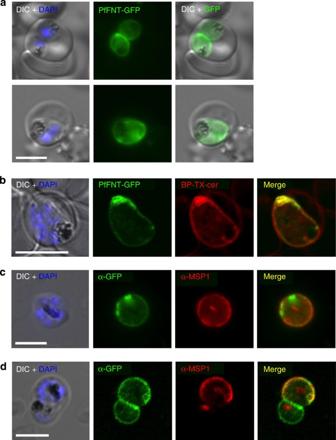Figure 4: Localization of PfFNT in infected erythrocytes. (a) Fluorescence pattern of live, PfFNT-GFP expressing early (top panel) and late trophozoites (bottom panel) within erythrocytes. DIC, differential interference contrast; DAPI (blue), nuclear stain; GFP (green). (b) A single confocal section through an infected erythrocyte. Bodipy-TX-ceramide (red), lipid membrane stain. (c,d) Co-localization in the plasma membrane of PfFNT-GFP with merozoite surface protein 1 (MSP1) by fluorescence microscopy (c) or a single confocal section (d) using anti-GFP and anti-MSP1 antibodies. Scale bars, 5 μm. Figure 4: Localization of PfFNT in infected erythrocytes. ( a ) Fluorescence pattern of live, PfFNT-GFP expressing early (top panel) and late trophozoites (bottom panel) within erythrocytes. DIC, differential interference contrast; DAPI (blue), nuclear stain; GFP (green). ( b ) A single confocal section through an infected erythrocyte. Bodipy-TX-ceramide (red), lipid membrane stain. ( c , d ) Co-localization in the plasma membrane of PfFNT-GFP with merozoite surface protein 1 (MSP1) by fluorescence microscopy ( c ) or a single confocal section ( d ) using anti-GFP and anti-MSP1 antibodies. Scale bars, 5 μm. Full size image The characteristics of PfFNT L -lactate transport (expression profile, low-affinity and high-capacity transport, substrate selectivity, inhibitory compound pattern and localization) reflect those obtained earlier with living parasites. Hence, it is quite possible that plasmodia express PfFNT as a single lactate transporter, comparable, for example, to the single aquaglyceroporin [25] . Deletion of the PfFNT gene, for which a conditional knockout system is likely to be required, will ultimately reveal its contribution to P. falciparum viability and virulence. It is particularly appealing that PfFNT is structurally unrelated to human transporters and that crystal data are available from homologous bacterial FNTs [12] , [13] , [14] , [15] , [16] , enabling development of lactate transport as a novel antimalarial drug target. Conversely, the identification of PfFNT inhibitors may aid development of antibiotics. In fact, we were able to inhibit E. coli FocA by α-fluorocinnamate ( Supplementary Fig. 14 ). Future steps will involve elucidation of the PfFNT crystal structure and expansion of the pool of FNT inhibitor compounds using phloretin/furosemide/cinnamate as leads to increase specificity and potency. Microbial strains Yeast strains used in this study were for monocarboxylate and malonate transport assays W303-1A Δjen1 Δady2 (MATa, can1-100, ade2-1 oc , his3-11-15, leu2-3,-112, trp1-1-1, ura3-1, jen1::kanMX4, ady2::hphMX4 ) [19] kindly provided by M. Casal, and for glycerol transport assays BY4742Δfps1 (MATa, his3-1, leu2Δ0, lys2Δ0, ura3Δ0, fps1::kanMX ) [32] obtained from Euroscarf. For PfFNT localization P. falciparum strain 3D7 was used [10] . Sequence analysis, topology plots and expression profiles Protein sequences were derived from PlasmoDB [7] and the NCBI protein database; protein structure data were from RCSB protein data bank. Sequence alignments were carried out using the clustalw algorithm and hand-adjusted if necessary. Alignments and topology plots were set with TeXshade and TeXtopo, respectively. Sequence identity and similarity was calculated with TeXshade. Protein structures were plotted with the pymol software. Expression profiles were retrieved from PlasmoDB from data on the P. falciparum transcriptome during intraerythrocytic development. Therefore, synchronized parasites had been assayed by RNA sequencing at eight time points during the infected red blood cell cycle, see ref. 11 for details. Expression plasmids, yeast transformation and culture P. falciparum 3D7 total RNA, provided by I. Bruchhaus, was transcribed into cDNA for amplification of PfFNT, PFB0465c and PFI1295c. PCR products were subcloned into the yeast expression vector pDR196 (Addgene) encoding an N-terminal haemagglutinin epitop and a C-terminal His 10 -tag. After codon analysis, optimized constructs were synthesized (>39% GC, Geneart/Lifetechnologies). The coding region of the yeast endogenous lactate transporter Jen1 was amplified from Saccharomyces cerevisiae BY4742 genomic DNA and ligated into pDR196. The pDR196-PfAQP construct and the yeast transformation protocol were described earlier [32] . All constructs were sequenced for verification. Transformed yeast was grown at 30 °C in synthetic selective media (s.d.) containing the appropriate nutritional requirements and 2% (wt/vol) glucose. Biotinylation of yeast surface proteins and western blot Yeast protoplasts were prepared to remove the cell wall and to enable access of the biotinylation agent to the plasma membrane. Therefore, 200 ml of yeast culture were grown to an OD 600 around 0.8, harvested (5 min at 4,000 g ), washed with water and subsequently washed with and resuspended in 4 ml buffer (50 mM KH 2 PO 4 , pH 7.2 (KOH), 0.2% β-mercaptoethanol). The suspension was incubated at 30 °C for 15 min shaking at 90 r.p.m. Two milligrams zymolyase 20 T (MP Biomedicals), 200 mg BSA and 8 ml sucrose buffer (50 mM KH 2 PO 4 , pH 7.2 (KOH), 0.2% β-mercaptoethanol and 1.8 M sucrose) were added and incubated at 30 °C for 1 h shaking at 90 r.p.m. Protoplasts were collected at 900 g for 5 min, washed and resuspended in 4 ml stabilizing sorbitol buffer (10 mM MOPS, pH 7.2 (NaOH), 50 mM NaCl, 5 mM CaCl 2 and 1.2 M sorbitol). N-hydroxy-succinimide-activated biotin with a disulfide linker, sulfo-NHS-SS-biotin (Pierce), was used for biotinylation according to the manufacturer’s protocol. Briefly, 6 mg of sulfo-NHS-SS-biotin were dissolved in 8 ml PBS, added to 3 ml of the protoplast preparations and incubated on ice for 1 h. Protoplasts were collected (900 g , 10 min) and washed three times with TRIS-buffered saline, TBS. Protoplast disruption was carried out in 2 × 1 ml TBS (with protease inhibitor cocktail) by repeated vortexing with acid-washed glass beads. Cell debris was removed at 1,000 g , 5 min, 4 °C. Biotinylated surface proteins were extracted from the supernatant by incubation with 500 μl NeutrAvidin agarose suspension (Pierce) at room temperature for 1 h on a rotator. Bound diotinylated protein was released by reducing the disulfide bond in the biotin-linker using 200 μl PBS supplemented with 50 mM dithiothreitol for 1 h at room temperature on a rotator. The procedure of protoplastation, biotinylation and surface protein extraction picked up only 1% of intracellular protein as tested with yeast expressing green fluorescent protein, GFP, versus a positive control, that is, the plasma membrane residing, plasmodial aquaglyceroporin, PfAQP [25] ( Supplementary Fig. 11 ). Extracted surface proteins were separated using SDS–PAGE, transferred to PVDF membranes and probed with a monoclonal anti-haemagglutinin antibody (Roche) and a horseradish peroxidase-linked secondary antibody (Jackson ImmunoResearch) for detection using ECL plus (GE Healthcare) and documentation with a Lumi-Imager F1 (Roche). Phenotypic growth assays Yeast cells were harvested (5 min at 4,000 g ) in the exponential phase at an OD 600 of ~0.8, washed twice with water and resuspended in water. For growth assays on solid agar media, yeast suspensions were diluted to an OD 600 of 1 (±10%) and 5 μl of serial tenfold dilutions were spotted on s.d. agar media with 2% glucose (control) or 0.25% L -lactate (assay), pH 5.6 (20 mM 2-( N -morpholino)ethanesulfonic acid MES). The plates were incubated at 30 °C for 5 days. For growth assays in liquid media, the yeast suspensions were diluted to an OD 600 of 2 (±25%) and 10 μl of cell suspension was added to 290 μl of liquid s.d. media with 0.25% L -lactate. The media were buffered to pH 4.0 and 5.0 (25 mM succinate), pH 6.0 (20 mM MES) or pH 7.0 and 8.0 (50 mM TRIS). Growth was determined for 160 h in multiwell honeycomb microplates as turbidity at 420–580 nm (Bioscreen C, Oy) and the area under the curve was calculated [33] . Direct transport assays using radiolabelled substrates The protocol was adapted from ref. 34 . Yeast suspensions of an OD 600 of 50 (±10%) were prepared in 50 mM HEPES/TRIS, pH 6.8 and kept on ice. Other pH conditions were established if required using 50 mM HEPES/TRIS (pH 7.8), 50 mM MES/TRIS (pH 5.8) or 50 mM citric acid/TRIS (pH 4.8, 3.8 and 2.8). The assays were carried out with at least three replicates at 18 °C in 1.5 ml reaction tubes containing 80 μl aliquots of yeast suspension. Uptake of L -lactate was initiated by adding 20 μl of L -lactate solution to yield a final concentration of 1 mM L -lactate and 0.02 μCi radiolabelled L -[1- 14 C]-lactate (other concentrations and radiolabelled substrates as indicated). The reaction was stopped at defined time points by rapid dilution with 1 ml of ice-cold water and transferred on a vacuum filtration unit fitted with a GF/C filter membrane (Whatman). The cells were washed once with 7 ml ice-cold water. Dilution, filtration and washing were accomplished within less than 10 s, and any loss of radiolabelled substrate from the cells during the procedure was within the error margin of the method itself as determined by an experiment in which an isomolar 1-mM substrate solution (without radiolabel) was used for dilution and washing. Any osmotic effect due to addition of compounds to the external buffer is compensated within a few seconds by the water permeability of the yeast plasma membrane and, thus, does not interfere with the transport assays [32] . The filter membranes were transferred to scintillation vials containing 5 ml of scintillation fluid (Quicksafe A, Zinsser Analytic) and analysed using a Packard TriCarb liquid scintillation counter (PerkinElmer Inc.). For chemical modification of solvent-accessible histidines, 1 mM DEPC (Sigma-Aldrich) from a freshly prepared stock solution in anhydrous ethanol was added to the yeast suspension 10–15 min before the transport assay. The final ethanol concentration of 1% did not affect transport. Proton decoupling was achieved by addition of 1 mM 2,4-dinitrophenol (from a 100-mM stock in 70% ethanol; Sigma-Aldrich) or 50 μM carbonylcyanide-3-chlorophenylhydrazone (from a 50-mM stock solution in 70% ethanol; Sigma-Aldrich) to the cell suspension 5–10 min before the experiment. The inhibitory potential of phloretin, furosemide, cinnamic acid derivatives and pCMBS on the L -lactate uptake via PfFNT was tested by pre-incubation of the yeast suspensions for 10–20 min with these compounds (Sigma-Aldrich). Depending on the solubility, stock solutions were made with buffer (50 mM HEPES/TRIS, pH 6.8), 70% ethanol or DMSO. The DMSO concentration in the assay never exceeded 3%, which showed to have an inhibitory effect itself of 13±1.2%. The obtained data were corrected accordingly. For testing substrate transport of PfFNT in the efflux direction, 80 μl suspension aliquots of yeast cells were preloaded by adding 20 μl of L -lactate or formate solution for 4 min or for 8 min in the case of D -lactate to yield a final concentration of 1 mM substrate and 0.02 μCi radiolabelled 14 C substrate. To minimize metabolic conversion of D -lactate by three endogenous yeast D -lactate dehydrogenases, respective cells were additionally treated with 0.5% deoxy- D -glucose and cooled to 0 °C. The cells were collected by centrifugation and 90 μl of supernatant were removed. To initiate substrate export, the external solution was diluted by a factor of 100 by resuspending the cells in 1 ml substrate-free buffer of 50 mM HEPES/TRIS, pH 6.8. Substrate efflux was terminated at defined time points by vacuum filtration of the cell suspension through a GF/C filter membrane (Whatman) and washing with 7 ml ice-cold water. Determination of external pH shifts due to lactate uptake Yeast cells were grown to an OD 600 of 1 (mid-log phase), collected with centrifugation at 4,000 g for 5 min at room temperature and washed twice with deionized water. Cells were resuspended in deionized water to an OD 600 of 60. One millilitre of the cell suspension was diluted into 7 ml of weakly buffered incubation solution (4 mM MES/triethanolamine, pH 5.1, 0.5% deoxy- D -glucose). The pH of the external buffer was recorded at intervals of 10 s by using a SenTix950 pH electrode connected to a Multi9310 pH meter (WTW GmbH, Germany). After equilibration for 5–10 min, uptake was initiated by addition of sodium L -lactate from a 1-M stock solution prepared in the same buffer. All measurements were carried out at room temperature. Reconstitution of PfFNT and stopped-flow lactate transport assay Codon-optimized PfFNT DNA was ligated into pIVEX2.4a (Roche Diagnostics). PfFNT protein was synthesized in an E. coli S30 extract-based, continuous exchange cell-free system containing 1% Brij 78 for solubilization [35] . The reaction was sustained by 17 volumes of feeding mix. PfFNT was bound to Ni-NTA and eluted using increasing concentrations of imidazole (20–500 mM) in purification buffer (20 mM Tris-HCl, 150 mM NaCl, 0.05% Brij 78). For proteoliposome preparation [36] E. coli polar lipids (Avanti Polar Lipids) were dissolved in chloroform to 25 mg ml −1 , evaporated in a nitrogen stream and hydrated in 2 mM 2-mercaptoethanol to a final concentration of 50 mg ml −1 for 1 h at room temperature. Hundred microlitres of lipid solution plus 10 μl of preparation buffer (20 mM HEPES, pH 6.8) were sonicated for 45 min in a nitrogen atmosphere. Then, 100 μg of solubilized PfFNT (0.05% Brij 78 final concentration) was added and the mixture was incubated on ice for 30 min. The detergent was diluted by injection into 25 volumes of preparation buffer, the resulting suspension was kept at room temperature for 20 min and proteoliposomes were harvested by centrifugation (140,000 g for 45 min). The proteoliposomes were resuspended in preparation buffer to 26 μg ml −1 PfFNT. Lactate transport was assayed using a stopped-flow apparatus (SFM-3, Bio-Logic) [12] . The proteoliposomes were rapidly mixed at 20 °C with an equal volume of preparation buffer supplemented with 20 mM L -lactate to yield a 10-mM inward lactate gradient. In an initial, rapid phase the proteoliposomes shrank due to osmotic water efflux, followed by a second, slower phase of lactate influx. Changes in proteoliposome volume was monitored as changes in 90° light scattering at 546 nm (ref. 12 ). Localization of PfFNT in infected erythrocytes For expression of GFP-tagged PfFNT in P. falciparum parasites, the coding sequence was cloned into pARL1-PF08_0003-GFP via KpnI and AvrII replacing PF08_0003 (ref. 30 ). Parasites were cultured with O+ erythrocytes in RPMI 1640 plus 0.5% Albumax, transfected [37] , selected using 4 nM WR99210 (Jacobus Pharmaceuticals) and imaged with a Zeiss Axioskop M1 microscope at × 100/1.4 oil immersion [31] . Nuclei were visualized with 1 μg ml –1 of 4′,6-diamidino-2-phenylindole (DAPI, Roche). For confocal microscopy, infected red blood cells were labelled with 2.5 mM Bodypi-TR-C_5-ceramide for 30 min at 37 °C as described [31] and imaged with a Fluoview 1000 confocal microscope (Olympus) equipped with a × 100/1.4 oil immersion lens. Immunofluorescence assays for the MSP1 co-localization were carried out according to established procedures using fixation in 4% formaldehyde, 0.0075% glutaraldehyde in PBS [38] but with parasites coated on multiwell slides using concanavalin A [39] with the following modifications: before the primary antibody incubation the cells were blocked and permeablized with 3% BSA, 100 mM glycine, 0.2% Triton-X-100 in PBS for 1 h. Primary antibodies were applied in 3% BSA, 100 mM glycine in PBS overnight and secondary antibodies for 1 h in 3% BSA in PBS. Antibodies used were rabbit antimerozoite surface protein 1, MSP1, (1: 500), a kind gift of M. Blackman and mouse monoclonal anti-GFP (Roche; 1:500). Secondary antibodies were Alexa-Fluor 594 goat anti-rabbit and Alexa-Fluor 488 goat anti-mouse (Molecular Probes), both diluted 1:2,000. DAPI was included into the secondary antibody solution at 1 μg ml –1 . How to cite this article: Wu, B. et al . Identity of a Plasmodium lactate/H + symporter structurally unrelated to human transporters. Nat. Commun . 6:6284 doi: 10.1038/ncomms7284 (2015).